Experimental demonstration of quantum digital signatures using phase-encoded coherent states of light Digital signatures are frequently used in data transfer to prevent impersonation, repudiation and message tampering. Currently used classical digital signature schemes rely on public key encryption techniques, where the complexity of so-called ‘one-way’ mathematical functions is used to provide security over sufficiently long timescales. No mathematical proofs are known for the long-term security of such techniques. Quantum digital signatures offer a means of sending a message, which cannot be forged or repudiated, with security verified by information-theoretical limits and quantum mechanics. Here we demonstrate an experimental system, which distributes quantum signatures from one sender to two receivers and enables message sending ensured against forging and repudiation. Additionally, we analyse the security of the system in some typical scenarios. Our system is based on the interference of phase-encoded coherent states of light and our implementation utilizes polarization-maintaining optical fibre and photons with a wavelength of 850 nm. Alice and Bob have become two of the most important figures in the science of information security, where Alice typically takes the role of sender and Bob receiver. To ensure the validity of important communications, Alice wants to transmit a message to Bob in such a way that he can verify that the message came from her and was not altered in transmission. Additionally it is required that a message that has been validated by one party is further validated by all other parties it is forwarded to. Modern information networks make extensive use of digital signatures to verify the origin and authenticity of messages. These digital signatures are typically based on so-called ‘trapdoor one-way functions’ used in public key cryptography [1] , [2] , [3] , which are easy to perform one way but computationally intensive to reverse without prior information. This prior information forms what is known as a ‘private key’, kept secret by Alice and used to decrypt information encrypted using her publicly available ‘public key’. However, there is currently no known proof that reversing such trapdoor one-way functions without the prior information will always be computationally intensive [4] and future advances in mathematical or computer science [5] , [6] may lead to insecurities in such approaches. Indeed, given enough computational resources the cryptosystem can be broken with current technology [7] , [8] , [9] . In contrast, quantum digital signatures (QDS) offer security verified by information-theoretical limits and quantum mechanics [10] , [11] . QDS is, roughly speaking, a quantum version of the Lamport public key based scheme for digital signatures [10] , [12] . In a digital signature scheme, it is vital not only that the public key reveals limited information about the private key, but also that the recipients of the public key can be sure that they have the same public key in order to prevent repudiation of a signature. Classical public keys are readily verified to be identical. Comparing quantum systems, however, is nontrivial [13] , [14] and in general difficult to implement [10] . In QDS, security against forging of a message either by Bob or Charlie, or by a fourth external party, is guaranteed as Alice alone has full knowledge about the quantum signature states. Security against repudiation by Alice, in other words that Bob and Charlie will agree on the validity of a forwarded message, is realised, roughly speaking, by ensuring that they have identical quantum signatures. The system must also be robust, implying that if all parties act as prescribed by the protocol, classical messages sent from Alice to any single recipient will be confirmed as authentic, except with negligible probability in the presence of realistic (experimental) imperfections in equipment. Also, if the authenticated message is forwarded, the message’s authenticity will be confirmed except with negligible probability. In our system, the signatures are encoded as the relative phase shifts of coherent states of light [15] . Quantum comparison of coherent states may be implemented using a 50:50 beamsplitter and has a higher success probability than general comparison methods [16] . Our experimental setup provides a method for two parties (Bob and Charlie) to receive quantum signatures, which serve as analogues to the public keys in classical cryptography schemes, from an untrusted Alice. These signature states are then used for the full QDS protocol. This allows Alice to sign a message so that it can be validated by Bob and/or Charlie. If an accepted message is forwarded, for example, from Bob to Charlie, then the forwarded message is guaranteed to also be accepted by Charlie as genuinely coming from Alice. 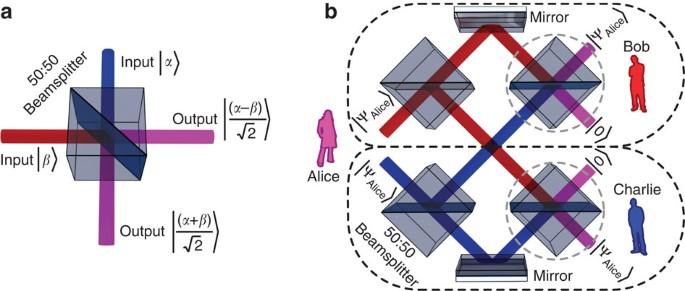Figure 1: Basic principles of our quantum digital signature scheme. (a) Field mixing on a 50:50 beamsplitter cube. The states |α〉 and |β〉 are coherent states15,17. (b) Quantum digital signature distribution in the case where Alice (the sender) is not trusted. Bob (one of the receivers) separates half of each signature state received from Alice using a beamsplitter, and sends it to Charlie, where it is compared with the signature half Charlie received from Alice using the 2nd beamsplitter within the grey dashed lines. Likewise, Bob compares the signature state he received directly from Alice with the one received via Charlie. The final beamsplitters in the dashed grey circles work as depicted inFig. 1a. Principles of QDS Figure 1 a shows how two coherent states of light mix on a 50:50 beamsplitter [17] . A coherent state | α 〉 is a quantum state, which closely resembles a classical electromagnetic wave. In mathematical terms, ā| α 〉= α | α 〉, where ā is the annihilation operator for the relevant electromagnetic field mode, and α is a complex number. The input states to the beamsplitter are | α 〉 and | β 〉 and the output states and . Clearly if α = β then , the vacuum state, and no light exits through that port. This simple operation forms the basis of the multiport signature comparison system employed by Bob and Charlie, shown in Fig. 1b . At each receiver the signature from Alice is split into two equal-amplitude components, and one of these is shared with the other receiver, who does the same to their copy of the signature. The retained component of the signature is then mixed on a beamsplitter with the component transmitted from the other receiver. It can be seen from Fig. 1a that if the two components are the same, then the original signature will be recovered through one port of the beamsplitter, and |0〉 will be generated at the other. For any other input state, the multiport renders the individual out-bound signature state symmetric with respect to Bob and Charlie. Recall, in order to repudiate a message, Alice has to cause a disagreement between Bob and Charlie concerning the validity of her message. As the states exiting the multiport are symmetric with respect to Bob’s and Charlie’s systems, Bob and Charlie’s measurement results will obey the same statistics, and thus if one party validates, so will the other. This is explained in more detail later. Figure 1: Basic principles of our quantum digital signature scheme. ( a ) Field mixing on a 50:50 beamsplitter cube. The states | α 〉 and | β 〉 are coherent states [15] , [17] . ( b ) Quantum digital signature distribution in the case where Alice (the sender) is not trusted. Bob (one of the receivers) separates half of each signature state received from Alice using a beamsplitter, and sends it to Charlie, where it is compared with the signature half Charlie received from Alice using the 2nd beamsplitter within the grey dashed lines. Likewise, Bob compares the signature state he received directly from Alice with the one received via Charlie. The final beamsplitters in the dashed grey circles work as depicted in Fig. 1a . Full size image To utilize the QDS protocol, Alice randomly selects a series of quantum states | αe iθ 〉 where α is fixed, θ ∈ {2 πp / N , p =0, 1, …, N −1}, and N is the number of possible phase encodings. The phase of each state is analogous to the classical private key. The principles of quantum mechanics prohibit determining the phases of the states, that is, the private key, with complete certainty if we only have access to the quantum state [14] , [18] . Each message bit is signed using a key of length L . For a one-bit message m , either 0 or 1, Alice generates two sets of phase-encoded states, with randomly chosen phases defining the corresponding private keys. Alice sends one copy of the pair of sets to Bob and one to Charlie. Bob and Charlie pass the complete series of encoded states { ρ 0, k } k and { ρ 1, k } k through the multiport of Fig. 1b . If the original signature states were identical coherent states, this operation will preserve them, otherwise it will symmetrize the overall state shared by Bob and Charlie, which prevents repudiation by Alice. Bob and Charlie then store their phase-encoded states in a quantum memory [19] . Quantum memories are a relatively immature technology [20] and have yet to demonstrate long-term storage of quantum states. In our experimental system, Bob and Charlie measure the phase of the laser pulses immediately after they have left the multiport. In the general case, to send a signed message, Alice sends the message and the classical description of the corresponding private key states to Bob (for example). Bob checks the classical description of the key states against those stored in his memory as follows. He generates coherent states according to Alice’s description, individually interferes them with the corresponding states in his memory, and checks whether the number of photodetection events at the signal null-port is smaller than s a L , in which case the message is confirmed to be valid. The fraction s a is called the authentication threshold. Alice must share a well-defined phase reference with all of the receivers to ensure that their measurement of her phase encodings is correct. Our experimental system time multiplexes the encoded signal and delayed reference pulse in one fibre. The exact mechanism is outlined in the Methods. Assuming that the authenticity of the message has been confirmed, Bob can then prove to Charlie that he has received that particular signed message from Alice. To do this, he forwards the message and the classical description of the signature states corresponding to the message he received from Alice to Charlie. To verify a signed message forwarded by Bob, Charlie follows the same procedure as Bob, but with a modified threshold s v > s a , called the verification threshold. The difference in the thresholds s a and s v is required to ensure security against repudiation by Alice, depends on the parameters of our system and will be given later. Essentially, since Bob and Charlie have symmetric quantum signature states they will obtain the same measurement statistics. The gap between s a and s v ensures that Alice cannot make one of them accept and the other reject a message, except with vanishingly small probability. The choice of mean photon number per pulse | α | 2 for the coherent states emitted by Alice to each party depends on the number of possible phase encodings N and the signature length L . 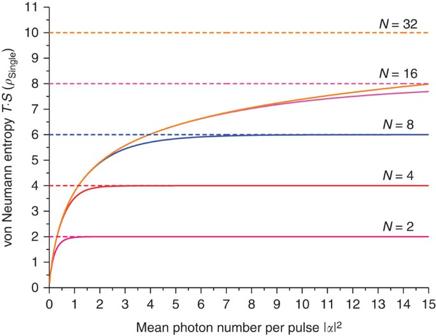Figure 2: Dependence of the von Neumann entropy for two receivers on mean photon number. The von Neumann entropyS(ρSingle) is shown scaled for two receivers (T=2). Five different possible numbers of phase encodingsNequal to 2, 4, 8, 16 and 32 are shown. The asymptotic value of the entropy increases with the number of phase encodingsN, indicating that it is possible to use higher mean photon numbers |α|2for greater values ofN. Figure 2 shows how the information about the phase of each encoded laser pulse, available to a malicious party, given by the von Neumann entropy [21] of the state ρ Single defined by: Figure 2: Dependence of the von Neumann entropy for two receivers on mean photon number. The von Neumann entropy S ( ρ Single ) is shown scaled for two receivers ( T =2). Five different possible numbers of phase encodings N equal to 2, 4, 8, 16 and 32 are shown. The asymptotic value of the entropy increases with the number of phase encodings N , indicating that it is possible to use higher mean photon numbers | α | 2 for greater values of N . Full size image varies with increasing | α | 2 , for two receivers ( T =2). In practice, we must ensure that the information about the whole signature known by Alice far exceeds that which is accessible to a malicious party with access to all signature states in circulation, that is, L ·log 2 ( N ) ≫ L · T · S ( ρ Single ). We will return to the issue of security below; a more detailed analysis is given in the Supplementary Discussion , where we find the optimal attacks and calculate the various cheating probabilities. It is an important assumption we adhere to that the channels from Alice to Bob’s and Charlie’s inputs to the multiport are under the control of the honest receiving parties, that is, an external party may not tamper with the states sent, although the channel is not assumed to be private. Otherwise a man-in-the-middle (impersonation) attack, where the attacker swaps Alice’s quantum signatures for their own, becomes possible. If authenticated quantum channels are presumed not to be available impersonation attacks possibly could be countered in a way similar to in quantum key distribution (QKD) as Alice is sending a restricted set of quantum messages. For this reason, in the more detailed security analysis, we have focused on the aspects of the QDS protocol that are genuinely different from the QKD setting. Schemes for either QKD or QDS that use linearly independent states, and which counter impersonation attacks through partial disclosure of key or signature states and discussion over an authenticated classical channel remain vulnerable to attacks using unambiguous state discrimination [22] . Such attacks, however, only place an upper bound on the total allowed loss. In our implementation, this bound is high and not of concern, as the success probability for an unambiguous measurement that distinguishes between all eight ideal quantum signature states is low, of the order of 10 −9 . 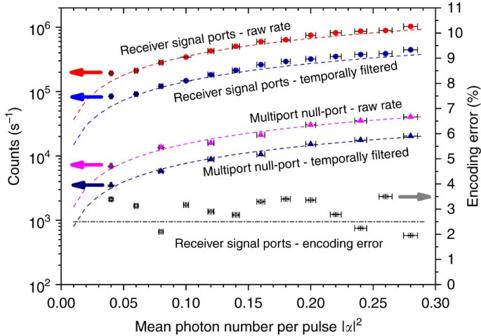Figure 3: Experimentally measured detector event count rates and encoding error for receiver Charlie. The system clock rate was 100 MHz and eight equally spaced phase encodings were used. Data points represent actual experimental results while dashed lines are theoretical predictions. The raw count rate is the detector click rate summed over both of Charlie’s signal SPADs after the demodulating interferometers. The time gated count rate is the raw count rate after temporal filtering using a 2 ns duration window centred on the expected arrival time to reduce the effects of background events, temporal intersymbol interference23and non-interfering photons. The encoding error is the number of temporally filtered detector events recorded by Charlie at the signal null-port divided by the total number of temporally filtered detector events he recorded. The experimental values have a square root uncertainty in count rate, while uncertainty in the mean photon number is dominated by a worst case scenario assumption than the pulse-to-pulse variance in the output power of our laser is the experimentally measured maximum of ±1.5%. Honest Alice Figure 3 shows the experimental results obtained by Charlie in the system using eight equally spaced phase encodings ( N =8) and an honest Alice sending the same signatures to both Bob and Charlie. For these measurements the phase modulator in the Alice to Bob fibre was deactivated. The dashed lines represent the predictions for the quantities using a theoretical model that is explained in more detail in the Methods, while the data points are actual experimentally recorded values. As the mean photon number per pulse launched by Alice into the comparison system increases, so the count rate at the detectors increases. The multiport null-port count rates are significantly lower than those at the signal port but are non-zero. The null-port counts are primarily owing to the interferometric fringe visibility of the multiport (although background events at the detectors do make a small contribution) [23] . This multiport null-port rate sets a baseline for the system operating with an honest Alice. The encoding error is defined as the number of temporally filtered pulses detected by a receiver at his signal null-port, divided by the temporally filtered total number of pulses recorded by that receiver. The encoding error rate is constant within experimental fluctuations across the range of experimentally examined values of | α | 2 , as the effects of intersymbol interference and background events in the detectors are negligible. Each of the six detectors has a mean dark-count rate of 320 counts per second, and the probability of temporal intersymbol interference for each detector is 3 × 10 −8 . Figure 3: Experimentally measured detector event count rates and encoding error for receiver Charlie. The system clock rate was 100 MHz and eight equally spaced phase encodings were used. Data points represent actual experimental results while dashed lines are theoretical predictions. The raw count rate is the detector click rate summed over both of Charlie’s signal SPADs after the demodulating interferometers. The time gated count rate is the raw count rate after temporal filtering using a 2 ns duration window centred on the expected arrival time to reduce the effects of background events, temporal intersymbol interference [23] and non-interfering photons. The encoding error is the number of temporally filtered detector events recorded by Charlie at the signal null-port divided by the total number of temporally filtered detector events he recorded. The experimental values have a square root uncertainty in count rate, while uncertainty in the mean photon number is dominated by a worst case scenario assumption than the pulse-to-pulse variance in the output power of our laser is the experimentally measured maximum of ±1.5%. Full size image Detection of discrepancies A necessary requirement for a system to be immune to Bob’s forgery is that Charlie is capable of detecting a discrepancy between Alice’s chosen phase encoding in a signature state and Bob’s average best guess of the phase. A discrepancy will cause a higher probability for a photodetection event on the signal null-port in the case when Charlie measures the pulse using a phase different from that actually encoded on the pulse. We experimentally verified this by looking at the encoding error at Charlie if he measures using a phase different from that defined by Alice. The results are shown in Fig. 4 . This allows us to characterize the effects of a mismatch between the encodings in true and forged quantum signatures. The off-diagonal elements correspond to Charlie measuring using a phase different from that used by Alice. The results show that Charlie can detect an increase in his encoding error percentage when Bob (or another external party) attempts to forge a message. A greater difference between the probabilities of null-port events for differing and identical phases reduces the required key length for a desired level of security. 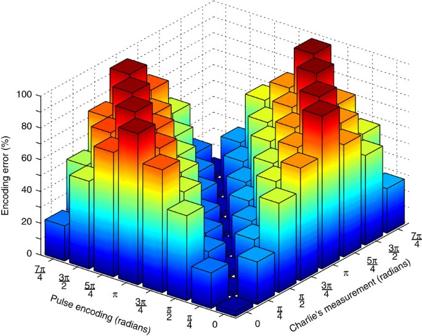Figure 4: Percentage encoding error for Charlie. The plot shows Charlie’s error encoding percentage when he measures using states with phases identical and different from those defined by Alice. The coherent states have mean photon number |α|2=0.16 and are chosen from a set ofN=8. Figure 4: Percentage encoding error for Charlie. The plot shows Charlie’s error encoding percentage when he measures using states with phases identical and different from those defined by Alice. The coherent states have mean photon number | α | 2 =0.16 and are chosen from a set of N =8. Full size image Certain types of malicious activities by Alice can also be detected by monitoring the multiport null-port count rates. We experimentally tested the case where Alice sends different signatures to Bob and Charlie. The phase modulator in the fibre connecting Alice to Bob was used to change the phase encoding of two pulses in every 16 by a fixed phase, and Charlie’s count rate at the multiport null-port and error rate were monitored. The results for the raw count rate at the multiport null-port can be seen in Fig. 5 . It can be observed from Fig. 5 that as Alice increases the magnitude of the phase difference between the states, the count rate at Charlie’s null-port increases as expected. 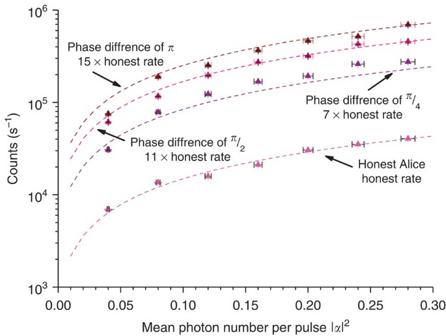Figure 5: Effect on the multiport null-port count rate if Alice sends different signature states to Bob and Charlie. Data points represent actual experimental results while dashed lines are theoretical predictions. She alters the phase encoding of two pulses in every 16 by a fixed amount. The ‘Honest rate’ is the observed multiport null-port count rate when Alice sends the same signature to Bob and Charlie. As Alice makes progressively greater changes to the phase encodings sent to one party, the count rate at the multiport null-port increases. It can be seen that a phase difference ofπ/4 increases the multiport null-port count rate by a mean factor of 7, a phase difference ofπ/2 increases it by a mean factor of 11 and a phase difference ofπincreases it by a mean factor of 15. The experimental values have a square root uncertainty in count rate, while uncertainty in the mean photon number is dominated by a worst case scenario assumption than the pulse-to-pulse variance in the output power of our laser is the experimentally measured maximum of ±1.5%. Figure 5: Effect on the multiport null-port count rate if Alice sends different signature states to Bob and Charlie. Data points represent actual experimental results while dashed lines are theoretical predictions. She alters the phase encoding of two pulses in every 16 by a fixed amount. The ‘Honest rate’ is the observed multiport null-port count rate when Alice sends the same signature to Bob and Charlie. As Alice makes progressively greater changes to the phase encodings sent to one party, the count rate at the multiport null-port increases. It can be seen that a phase difference of π /4 increases the multiport null-port count rate by a mean factor of 7, a phase difference of π /2 increases it by a mean factor of 11 and a phase difference of π increases it by a mean factor of 15. The experimental values have a square root uncertainty in count rate, while uncertainty in the mean photon number is dominated by a worst case scenario assumption than the pulse-to-pulse variance in the output power of our laser is the experimentally measured maximum of ±1.5%. Full size image A more careful security analysis can be found in the Supplementary Discussion , but will be outlined here. We identify two classes of forging attacks. In the active attack the malicious party (Bob or Charlie) is allowed to alter the states he forwards to the other party within the multiport to optimize his later cheating probability. In a passive attack, the recipients of the quantum signatures are benevolent throughout the signature distribution phase but will attempt to falsify a message later. This is a restricted setting, which corresponds to the case where each recipient is a priori equally likely to be the forger, or when a trusted third party holds the multiport. An external party, who does not hold any signature copies, will have a lower probability for successfully forging a message. The probability of cheating in a passive attack can be evaluated using the experimental results presented in Fig. 4 . This probability is also central to estimating the cheating probabilities using active attacks. To counter against active attacks, the outcomes at the multiport null-ports during signature distribution must be taken into account. In short, a low count rate at the multiport null-port guarantees that the probabilities of cheating using the active and passive attacks will not differ substantially. We now proceed to calculate the probability of cheating for a passive attack, saving the case of an active attack for the Supplementary Discussion . Assuming Bob is the forger, his optimal passive strategy for forging the message, say m =0, consists of producing a ‘best guess’ of the private key by inspecting his copy of the corresponding signature state and forwarding this guess to Charlie. We assume that the phases of the states have been generated independently and uniformly at random. Then Bob’s optimal strategy is to employ a single generalized measurement applied on each of the states in his signature. The probability of causing a photodetection event, when verifying a single state in the signature, is then given by where c φ,θ is the probability of a photodetection event in Charlie’s signal null-port arm, given that ρ θ is the coherent state sent by Alice, with phase θ , and the phase angle declared by Bob is φ . The operators Π φ describe the measurement made by Bob, on the signature copy or copies he has access to, to select the best possible phase angle φ . Bob’s optimal measurement, minimizing the probability to cause a photodetection event is a minimum cost measurement [18] , with the cost matrix C with elements c φ,θ . The cost matrix C is obtained experimentally for our system, and is related to the encoding error matrix shown in Fig. 4 . The cost matrix additionally takes into account vacuum events on the signal ports, which are not included in the calculation of the encoding error. The full cost matrix is given in the Supplementary Discussion . We assume that the states in both Bob’s and Charlie’s quantum signatures are perfect, without the loss of generality, as (random) imperfections could only degrade the probability of getting Charlie to accept a forgery. If Bob is honest then the maximum probability of causing a photodetection event is p original (equal to the largest diagonal element(s) of C ). In our experiment the diagonal elements of C exhibit a small standard deviation around a well-defined mean. As long as p forgery > p original , given a large enough sample size (that is, signature length L ), cheating and honest scenarios can be distinguished using statistical methods. For the values p forgery and p original , one may set the authentication and verification thresholds as s a =1/3 g+ p original and s v =2/3 g+ p original . The gap g = p forgery − p original appears as the central parameter of the cheating probabilities and is equal to 8.03 × 10 −4 ±0.3 × 10 −4 for our system. The probability of forging using a passive attack equals the probability of a cheating Bob causing fewer than s v L photodetection events in Charlie’s signal null-port arm. Using Hoeffding’s inequalities [24] , as outlined in the Supplementary Methods , we bound this as Analogously, the probability ɛ robustness , for Bob and Charlie to reject a message from Alice, if all parties are honest, is Without errors caused by imperfections in the components, honest Bob and Charlie would never reject a message from an honest Alice. For the derivation of the parameters above see the Supplementary Discussion . Further to the probability of forging a message, there also exists a probability of repudiation. To repudiate her signature, a malevolent Alice needs to prepare the signature states so that Bob accepts and yet Charlie rejects the message when Bob forwards it, or vice versa. For this purpose, she may send different signature states to Charlie and Bob, or more generally, she may use any type of 2 L mode states, including entangled and mixed states. However, regardless of her choice of states, assuming an ideal multiport, the signature states Charlie and Bob end up with are symmetric under the swap of Charlie and Bob’s systems. Thus, the probability matrix describing the a priori occurrence of photodetection events in Bob and Charlie is symmetric. To maximize the probability of causing a mismatch in Charlie and Bob, required for repudiation, the most Alice can achieve is that with probability 1/2, Charlie detects a photon and Bob does not, and with probability 1/2 the opposite. To ensure repudiation of the signature, the number of cases where Charlie detects photons and Bob does, or vice versa, needs to be higher than gL , and the probability of this happening is upper bounded by [10] , [16] ɛ repudiation =(1/2) gL /3 . Imperfections could increase the factor of 1/2 in ɛ repudiation . However, for our system this increase is such that ɛ repudiation is smaller than ɛ forging , and thus ɛ forging bounds the overall security of our system. The work detailed in this article is an experimental demonstration of the distribution of quantum signatures. This system could also be used to share quantum frames of reference, and may be applicable to further quantum information protocols and experiments [25] , [26] . The current system does not utilize any form of quantum memory and it would be desirable to combine it with some form of the same [20] , [27] , [28] , or find a way to circumvent this requirement completely. Other challenges include extending the distance between Bob and Charlie beyond the current ∼ 5 m. At present, the pulses from the other party’s half of the signature must arrive at the final beamsplitter cube at the same time as those from the party’s retained half of the signature. As the distance between Bob and Charlie is increased, so the delay in the paths for the retained portion must increase, and this leads to instabilities increasing the error rate. This could be alleviated by temporarily storing the retained portions in a short-term quantum memory. Currently, the system is designed to operate with two receivers and scaling it up to a greater number of receivers is an area for future research. It is possible to generalize the scheme using balanced multiports, as suggested by Andersson et al. [16] Furthermore, Andersson et al. [16] suggested that the multiports may be realised in a time-resolved fashion or using fibre couplers. The primary reason for the small g value is the low photon flux at the receiver’s detectors. Reducing the loss of the multiport from the current 7.5 dB would be desirable. It may be possible to replace the air-gaps with fibre stretchers but these can increase the quantity of fibre within the system and lead to reduced up-time. Additionally, reducing the loss of the system overall will reduce the signature length L required for a given level of security. With the current system parameters, for signature lengths L of the order of 5 × 10 6 pulses the bounds on the failure probability become non-trivial (and decay exponentially quickly from that point on). Increasing the clock rate, and therefore the transmission rate of the system, is consequently an obvious goal. The phase modulators, lasers and driving electronics, are all capable of clock-rates up to a maximum of 3.3 GHz. System implementation The experimental implementation of the QDS system is shown schematically in Fig. 6 . This system encodes phase onto highly attenuated laser pulses and compares two copies of the quantum signature, simultaneously symmetrizing the states, using the multiport. Finally, Bob and Charlie measure the phases of the pulses and detect the photons using silicon single-photon avalanche diodes (Si-SPADs) [29] . The addition of a phase modulator in the final section of fibre between Alice and Bob allows us to test the multiport performance when Alice tries to cheat by sending different signatures to different recipients. The air-gap in the other arm allows the transmission losses to be balanced between each arm so that the same | α | 2 value is launched to each recipient, and permits compensation for small path-length differences between the two launch arms; | α | 2 is defined after Alice’s phase modulator/air-gap at the inputs to the multiport. 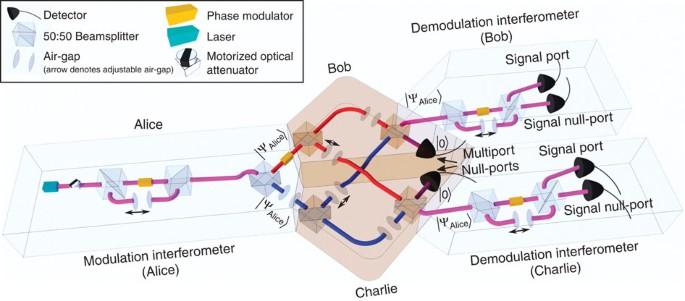Figure 6: Schematic diagram of the fibre-based experimental demonstration of quantum digital signatures. The laser used is a vertical cavity surface emitting laser (VCSEL) and the detectors are single-photon avalanche diodes (SPADs). The system is constructed from polarization-maintaining fibre to improve interferometric fringe visibility. The final phase modulator within Alice’s apparatus and corresponding adjustable air-gap can be used to test certain malicious activities implemented by Alice and are removed for experiments with honest parties. Figure 6: Schematic diagram of the fibre-based experimental demonstration of quantum digital signatures. The laser used is a vertical cavity surface emitting laser (VCSEL) and the detectors are single-photon avalanche diodes (SPADs). The system is constructed from polarization-maintaining fibre to improve interferometric fringe visibility. The final phase modulator within Alice’s apparatus and corresponding adjustable air-gap can be used to test certain malicious activities implemented by Alice and are removed for experiments with honest parties. Full size image To ensure a high interferometric fringe visibility in the interferometers of the system, it is necessary to ensure that the relative path-length differences remain constant to within a fraction of the emission wavelength of the source laser [30] . Adjustable air-gaps in active feedback loops are used to compensate for any slow time-dependent variations in the relative path lengths [23] . The fringe visibility is monitored during operation of the system and when a deviation from the expected value is obtained, signature distribution is halted and tuning carried out using a higher intensity signal with known phase modulation until the optimum visibility is obtained. Our interferometers had fringe visibilities of 98%. It is likely that the greatest contributions to the reduction in the visibility of the interferometers from 100% are owing to the linewidth of our laser source [30] and loss of polarization extinction ratio (PER) at non-ideal fusion splice and flat-polish bulkhead joins between the various fibres, which comprise the system. The stress members in the polarization-maintaining fibre must be aligned by eye during the splicing process, introducing human error and the flat-polish bulkhead connectors have variable misalignment because of manufacturing tolerances. The system has been assembled from polarization-maintaining fibre, which supports a single mode at a wavelength of 850 nm. The use of polarization-maintaining fibre ensures good fringe visibility in the interferometers of the system as high visibilities can be achieved when interfering two highly linearly polarized light fields [31] , and the use of a single spatial mode in the fibre reduces temporal broadening of the pulse. An operating wavelength of 850 nm was chosen to provide compatibility with comparatively mature high detection efficiency thick junction Si-SPADs [29] . The system operates at a pulse repetition frequency of 100 MHz to avoid intersymbol interference when using these detectors [29] . Si-SPADs were selected as detectors as the losses of the system (7.5 dB from the comparison stage input to each demodulation interferometer and 7.1 dB for each demodulation interferometer) mean that the pulses transmitted by Alice are in the single-photon regime at the detectors. Detectors of this type have been previously been used successfully in quantum information experiments [32] , [33] . The detection efficiency of the Si-SAPDs used for these experiments exhibits a count rate dependent variation. At higher count rates, the detection efficiency of the detectors decreases, reaching a minimum of 36.8% as opposed to the maximum value [34] of 42%. This system time multiplexes a phase reference pulse between successive 100 MHz clocked signal pulses using an asymmetric double Mach–Zehnder approach as used in many QKD systems employing phase basis sets [35] . In an ideal system, the receivers would utilize their paths with air-gaps to delay only the signal pulse so that it recombines with the corresponding reference, revealing the phase encoding. However, in a real system there will be photons, which take non-interfering paths in sender and receiver (that is, both short paths or both delayed paths) contributing nothing to the signature [35] and these are software gated from the photon arrival times recorded using the free-running Si-SPADs. In post-processing, the time gating software opens a window of duration 2 ns centred on the expected arrival time of a pulse and disregards events which occur outside of this window. Photon source characterization A vertical cavity surface emitting laser (VCSEL) [36] emitting at a wavelength of 849.8 nm, and with a spectral full-width at half maximum (FWHM) of 0.23 nm, was selected as the photon source in these experiments. In common with most other diode lasers, VCSELs exhibit a temperature dependent output wavelength [37] and consequently the VCSEL used in these experiments was mounted on a custom temperature controller and maintained at an operating temperature of 15±0.1 °C to ensure wavelength stability. The central wavelength of the laser had a measured wavelength shift of 77 pm per °C. The laser was driven using a 500-ps wide square electrical pulse at a repetition rate of 100 MHz using a commercial driving board, which ultimately produced optical output pulses of duration 780 ps FWHM. To improve the PER of the VCSEL [37] , it was necessary for the laser output to be transmitted through two high extinction ratio (in excess of 10,000:1) polarizers before being launched into the single-mode polarization maintaining fibre from which the main part of the optical system was comprised. The VCSEL output had a PER of 7:2 while for the light after the cleanup polarizers the PER was measured as being in excess of 1,200:1. Our measurement of the pulse-to-pulse variance of the output power of the VCSEL was limited by the resolution and noise level of our detector, but can be stated to be lower than 3%. The mean photon number per pulse | α | 2 was set using a computer-controlled motorized attenuator. A stepper motor drives a screw into or out of a collimated beam to provide the required attenuation. The motorized attenuator exhibits reproducibility of attenuation setting to within 1% of the calibrated value. In all uncertainty analyzes we have assumed a worst case scenario that the uncertainty in | α | 2 is dominated by the pulse-to-pulse variance in the output power of the VCSEL. The sender and receivers utilize phase modulators with a voltage to enact an optical phase change of π radians ( V π ) of 6 V. The driving electronics for the phase modulator have a pulse-to-pulse amplitude variance, which corresponds to a variance in the desired phase encoding of ±1.6 × 10 −3 radians or ±0.2% of the difference between successive values when 8 encodings are used. Theoretical modelling The theoretical model for the count rates is based on our previous work detailed in ref. 23 . The theoretical model requires knowledge of the system losses, clock rate (100 MHz), detector dark-count rate (320 counts per second), detector detection efficiency (42%), classical visibility (98%) and system instrument response function (modelled as the PerkinElmer thick junction silicon single-photon avalanche diodes of per ref. 23 ). To calculate the raw count rate at the receiver we model the multiport and receiver as losses of 7.5 and 7.1 dB, respectively, without taking into account interferometric visibility, as in equation (1) of ref. 23 . The temporally filtered count rate at the receiver was calculated following the same method as outlined in ref. 23 with the same instrument response function parameters. The encoding error was calculated using a modified form of the equations used to predict the quantum bit error rate. In equation (8) of ref. 23 the protocol-dependent scaling term ( α Protocol ) was set equal to unity so that the dark-count contribution was given by where υ is the clock frequency of the system (100 MHz), R Dark is the detector dark-count rate (320 counts per second), Δ T is the time gate duration (2 ns centred on the expected peak position) and R TimeGated (Δ T ) is the count rate remaining after temporal filtering by the 2 ns gate, as indicated by the triangular points on Fig. 3 . Calculation of the temporally filtered rates proceeded as in the case of ref. 23 . The raw count rates at the null, or vacuum state, ports of the multiport, were predicted by modelling the multiport as a loss of 7.5 dB and then utilizing the definition of visibility as (where I Max is the intensity of an interference maximum and I Min is the intensity of an interference minimum) with the count rates substituted for the intensities. For a visibility of 98% the theoretically predicted count rate at the signal output was substituted into the visibility equation as I Max and the equation rearranged to give I Min as the count rate on the multiport null-port. The theoretical model can be used to predict the results shown in Fig. 4 (and by extension the cost matrix C ) and Fig. 5 . The visibility is modelled using equation (6) above, equation (5) of ref. 23 and the cosine dependency of the phase sensitivity of a Mach–Zehnder interferometer given in equation (36) of ref. 38 . How to cite this article: Clarke, P.J. et al. Experimental demonstration of quantum digital signatures using phase-encoded coherent states of light. Nat. Commun. 3:1174 doi:10.1038/ncomms2172 (2012).